Dynactin functions as both a dynamic tether and brake during dynein-driven motility Dynactin is an essential cofactor for most cellular functions of the microtubule motor cytoplasmic dynein, but the mechanism by which dynactin activates dynein remains unclear. Here we use single molecule approaches to investigate dynein regulation by the dynactin subunit p150 Glued . We investigate the formation and motility of a dynein-p150 Glued co-complex using dual-colour total internal reflection fluorescence microscopy. p150 Glued recruits and tethers dynein to the microtubule in a concentration-dependent manner. Single molecule imaging of motility in cell extracts demonstrates that the CAP-Gly domain of p150 Glued decreases the detachment rate of the dynein–dynactin complex from the microtubule and also acts as a brake to slow the dynein motor. Consistent with this important role, two neurodegenerative disease-causing mutations in the CAP-Gly domain abrogate these functions in our assays. Together, these observations support a model in which dynactin enhances the initial recruitment of dynein onto microtubules and promotes the sustained engagement of dynein with its cytoskeletal track. Cytoplasmic dynein is the major microtubule minus-end directed motor in higher eukaryotes. Dynactin, a large multi-subunit protein complex, interacts with dynein and is essential for a broad range of cellular functions including organelle transport and mitotic spindle assembly [1] . Dynactin was first identified as an activator of dynein that increased the ability of dynein to transport organelles [2] but the mechanisms involved in dynein activation are not yet understood. Structurally, dynactin can be divided into two parts—an actin-like Arp1 rod that along with associated subunits forms the base of the complex and a projecting side arm formed from the dimerization of the largest subunit in the complex, p150 Glued (refs 3 , 4 ). p150 Glued interacts directly with the dynein intermediate chain (DIC) of the dynein motor [5] , [6] . p150 Glued also interacts with microtubules via its Cytoskeletal Associated Protein, Glycine-rich (CAP-Gly) domain at the N terminus [7] which is followed by a highly basic region that has a lower affinity interaction with microtubules [8] , [9] . In vitro motility studies using beads coated with purified proteins demonstrated that the microtubule-binding capacity of dynactin increases the processivity of mammalian dynein [8] , [10] . Despite these initial studies, the mechanisms by which dynactin enhances dynein-driven motility have remained controversial. For example, dynactin has been shown to enhance the processivity of yeast dynein, which differs from the mammalian motor in key biophysical properties including velocity and the frequency of backward stepping [11] . Surprisingly, however, the dynactin-dependent enhancement of the run lengths of yeast dynein in single molecule assays does not appear to require the CAP-Gly domain [12] , although at the cellular level this highly conserved domain contributes to the initiation and persistence of dynein-dependent nuclear movement [13] . Studies in higher eukaryotes also suggest that the CAP-Gly domain may be dispensable for some cellular functions, including the trafficking and localization of organelles in S2 and HeLa cells [14] , [15] . In contrast, both cellular and in vivo studies have demonstrated that the CAP-Gly domain of dynactin is essential for dynein function in neurons. In Drosophila and mammalian neurons, the CAP-Gly domain enhances the retrograde flux of cargoes from the distal axon [16] , [17] . An ordered recruitment pathway has been proposed, in which binding of dynactin to dynamic microtubules enriched in the distal axon leads to the enhanced recruitment of dynein, permitting the efficient initiation of retrograde transport [18] . Importantly, mutations in the CAP-Gly domain of p150 Glued cause human disease, including the motor neuron degenerative disease HMN7B and a lethal and rapidly progressive variant of parkinsonism known as Perry syndrome [19] , [20] . While the HMN7B-associated G59S mutation induces misfolding and aggregation [21] , the Perry syndrome mutations cause a loss of CAP-Gly function in cellular assays [17] . Together, these genetic findings indicate a key role for the CAP-Gly domain of dynactin in neurons in vivo . In light of these observations, we sought to develop a minimal in vitro system to more fully test the mechanisms by which dynactin activates dynein. Our data provide direct evidence that the CAP-Gly domain of dynactin recruits dynein onto microtubules and maintains association of the motor with its track. Our findings demonstrate that dynactin accomplishes this by increasing the landing frequency of dynein and decreasing the likelihood of detachment by functioning as a dynamic tether. Surprisingly, the CAP-Gly domain also acts as a brake to slow the dynein motor. We propose that these functions of dynactin become essential under specific cellular regimes, such as initiation of organelle transport in regions of the cell with low microtubule density, or maintenance of processive motility for cargos with few dynein motors bound, functions of particular importance in long distance cargo transport in neurons. Dynein–GFP switches between processive and diffusive motion To study the regulation of dynein by dynactin, we employed single molecule approaches, using a recently established knock-in mouse line [22] to isolate green fluorescent protein (GFP)-tagged dynein. The neuron-specific isoform of dynein intermediate chain, DIC1 is replaced with a DIC1–GFP–3xFLAG transgene under the control of the endogenous promoter ( Fig. 1a ). We purified GFP-labelled dynein from the brain tissue of these mice using microtubule affinity and ATP release followed by sucrose gradient centrifugation. DIC1–GFP incorporates efficiently into the dynein complex and interacts with co-purifying dynactin ( Fig. 1b ). Photobleaching analysis indicates the expected stoichiometry of two DIC1–GFP per dynein complex ( Supplementary Fig. 1a–c ). 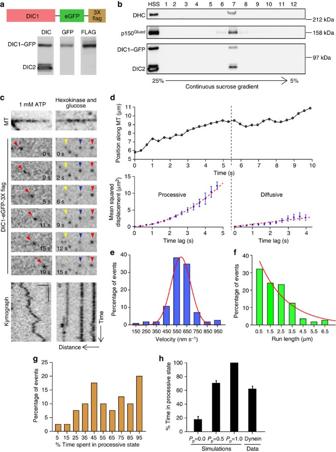Figure 1: Dynein–GFP switches stochastically from processive to diffusive states of motion. (a) Schematic of the DIC1–eGFP–FLAG gene knocked into the DIC1 locus. High speed supernatant (HSS) of homogenized mouse brain tissue was probed for DIC, GFP and FLAG. (b) Immunoblot analysis of sucrose gradient purified dynein. DIC1–GFP–FLAG is efficiently incorporated into the dynein complex as indicated by co-sedimentation with dynein heavy chain (DHC) at 20 S. (c) Time series and corresponding kymograph showing projection of the movement of the particle over time for a single dynein–GFP molecule at 1 mM Mg-ATP and in the presence of hexokinase and glucose (ATP depletion system). Horizontal bar, 2 μm. Vertical bar, 5 s. All the images are contrast inverted to represent the signal as black on a white background. (d) A representative trajectory of a dynein–GFP molecule. Following gradient analysis for node detection (see Methods), mean-squared displacement (MSD) analysis shows that the motion switches from processive (MSD=v2t2) to a diffusive state (MSD=2Dt). Error bars indicate s.e.m. (e,f) Distributions of velocities and run lengths of particles tracked (n=112, three independent experiments). Curves represent a Gaussian distribution and an exponential decay curve respectively. (g) Frequency distribution for the amount of time the particles (n=40, two independent experiments) spent in a processive state. On average, about 60% of the time, the motion is processive. (h) Quantitation of the per cent time spent in processive state for simulated tracks alongside the average for experimental data obtained fromFig. 1g. Mean±s.e.m.n=50 for the simulations andn=40 for the experimental data. Figure 1: Dynein–GFP switches stochastically from processive to diffusive states of motion. ( a ) Schematic of the DIC1–eGFP–FLAG gene knocked into the DIC1 locus. High speed supernatant (HSS) of homogenized mouse brain tissue was probed for DIC, GFP and FLAG. ( b ) Immunoblot analysis of sucrose gradient purified dynein. DIC1–GFP–FLAG is efficiently incorporated into the dynein complex as indicated by co-sedimentation with dynein heavy chain (DHC) at 20 S. ( c ) Time series and corresponding kymograph showing projection of the movement of the particle over time for a single dynein–GFP molecule at 1 mM Mg-ATP and in the presence of hexokinase and glucose (ATP depletion system). Horizontal bar, 2 μm. Vertical bar, 5 s. All the images are contrast inverted to represent the signal as black on a white background. ( d ) A representative trajectory of a dynein–GFP molecule. Following gradient analysis for node detection (see Methods), mean-squared displacement (MSD) analysis shows that the motion switches from processive (MSD= v 2 t 2 ) to a diffusive state (MSD=2 Dt ). Error bars indicate s.e.m. ( e , f ) Distributions of velocities and run lengths of particles tracked ( n =112, three independent experiments). Curves represent a Gaussian distribution and an exponential decay curve respectively. ( g ) Frequency distribution for the amount of time the particles ( n =40, two independent experiments) spent in a processive state. On average, about 60% of the time, the motion is processive. ( h ) Quantitation of the per cent time spent in processive state for simulated tracks alongside the average for experimental data obtained from Fig. 1g . Mean±s.e.m. n =50 for the simulations and n =40 for the experimental data. Full size image We performed single molecule motility assays ( Fig. 1c , Supplementary Movie 1 ) and gliding assays ( Supplementary Fig. 1d ) to confirm that isolated dynein–dynactin complexes are functional. We observed processive, bi-directional ATP-dependent runs along the length of microtubules ( Fig. 1c ). These runs are punctuated by frequent directional switches as well as periods of apparent diffusion. While single dynein motors often diffuse along microtubules, two to three dyneins working together exhibit robust minus-end directed motility [23] , [24] as supported by our gliding assays with isolated dynein–dynactin complexes ( Supplementary Fig. 1d ). This behaviour may be a functional consequence of the flexible structure of the dynein motor, and may permit multiple dynein motors bound to a single cargo to function effectively in cells [25] , [26] . To examine the single molecule behaviour of dynein in more detail, we developed an algorithm (Gradient Analysis for Node Detection (GrAND)) to parse out these different states (see Methods). A given trajectory is first split into constant-velocity segments by gradient analysis and then mean-squared displacement (MSD) analysis is performed to classify each segment as processive or diffusive/confined. An example trajectory is shown in Fig. 1d . This trajectory was segmented using the GrAND method followed by MSD analysis, which indicated that the particle exhibited uniform processive motion in the first few seconds and then switched to diffusion for the last few seconds of the track ( Fig. 1d ). We performed this analysis on all the particles tracked and obtained velocities and run lengths from all processive segments. The resulting data are well fit by a Gaussian distribution and a single exponential decay curve ( Fig. 1e,f ). We also generated a frequency distribution for the fraction of time spent in processive state for all particles tracked ( Fig. 1g ). We observed that ~20% of the particles exhibited processive movement throughout their time bound to the microtubule. For the remainder of the particles, ~60% of their time bound to the microtubule was spent in a processive state; we did not observe a correlation between track duration and fraction of time spent in processive motion. To validate our method of analysis, we simulated particle motion using parameters from our experimental data (see Methods) and tested our algorithm in three scenarios—purely diffusive motion, purely processive motion and a mix of diffusive and processive motion with a 50% probability for either type, using concatenated track segments to fully model the stochastic switching observed for dynein ( Supplementary Fig. 1e ). Analysis of the simulated data indicated that our method was robust for fully processive motion. We observed a false-positive detection rate of ~20% for purely diffusive motion ( Fig. 1h ), that reduced to ~10% if we modelled continuous rather than segmented tracks. However, to more closely represent the motility of dynein, we focused on simulations with track segments (see Methods). Importantly, the intermediate condition of mixed motility was determined to be processive ~70% of the time, which is in close agreement with our experimental data. p150 Glued enhances dynein recruitment onto microtubules To dissect the role of dynactin in dynein-driven motility, we generated a recombinant human p150 Glued 1-CC1 construct fused to C-terminal Halo and FLAG tags, expressed and purified from insect cells. This construct includes the N-terminal tandem CAP-Gly and basic microtubule-binding domains followed by the first coiled-coil (CC1) domain that binds dynein ( Fig. 2a,b ). The 1-CC1 construct lacks the C-terminal domains of p150 Glued that mediate association with the Arp1 filament [7] and which are not soluble when expressed recombinantly (ref. 27 and our unpublished observations). We purified the construct using FLAG affinity chromatography followed by labelling with a tetramethylrhodamine (TMR) dye that binds irreversibly to the Halo tag ( Fig. 2c ). The 1-CC1 fragment of p150 Glued is sufficient to bind dynein ( Supplementary Fig. 2a ). Single molecule assays on immobilized microtubules demonstrate microtubule-binding activity, with p150 Glued 1-CC1-TMR exhibiting lattice diffusion along the length of the microtubule ( Fig. 2d ). 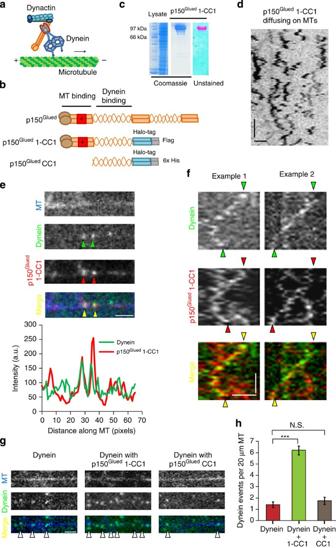Figure 2: p150Gluedco-migrates with dynein and enhances its recruitment onto microtubules. (a) Schematic illustrating the interaction of dynein with dynactin. (b) Schematic of the recombinant constructs p150Glued1-CC1 and p150GluedCC1 engineered with a Halo tag and affinity tags at the C terminus. (c) Coomassie-stained gel showing the lysate and the protein p150Glued1-CC1 after the final purification step. The unstained gel shows the labelling of the protein with TMR. (d) Contrast inverted kymograph of p150Glued1-CC1 diffusing on microtubules. Horizontal bar, 2 μm. Vertical bar, 5 s. (e) Co-localization of dynein and p150Glued1-CC1 on microtubules and corresponding line-scan intensity profile. (f) Representative kymographs of co-migration of dynein with p150Glued1-CC1. Horizontal bar, 2 μm. Vertical bar, 10 s. (g) Addition of p150Glued1-CC1 increases the landing events of dynein while p150GluedCC1 has no effect on the recruitment of dynein. Horizontal bar, 2 μm. (h) Quantitation of the landing events of dynein in each condition shows that p150Glued1-CC1 increases the landing events greater than fourfold. Mean±s.e.m.,n=25, two independent experiments, ***P<0.001, one-way analysis of variance with Tukey’spost-hoctest. Concentration of the recombinant protein used in each case is 4.5 nM. N.S., not significant. Figure 2: p150 Glued co-migrates with dynein and enhances its recruitment onto microtubules. ( a ) Schematic illustrating the interaction of dynein with dynactin. ( b ) Schematic of the recombinant constructs p150 Glued 1-CC1 and p150 Glued CC1 engineered with a Halo tag and affinity tags at the C terminus. ( c ) Coomassie-stained gel showing the lysate and the protein p150 Glued 1-CC1 after the final purification step. The unstained gel shows the labelling of the protein with TMR. ( d ) Contrast inverted kymograph of p150 Glued 1-CC1 diffusing on microtubules. Horizontal bar, 2 μm. Vertical bar, 5 s. ( e ) Co-localization of dynein and p150 Glued 1-CC1 on microtubules and corresponding line-scan intensity profile. ( f ) Representative kymographs of co-migration of dynein with p150 Glued 1-CC1. Horizontal bar, 2 μm. Vertical bar, 10 s. ( g ) Addition of p150 Glued 1-CC1 increases the landing events of dynein while p150 Glued CC1 has no effect on the recruitment of dynein. Horizontal bar, 2 μm. ( h ) Quantitation of the landing events of dynein in each condition shows that p150 Glued 1-CC1 increases the landing events greater than fourfold. Mean±s.e.m., n =25, two independent experiments, *** P <0.001, one-way analysis of variance with Tukey’s post-hoc test. Concentration of the recombinant protein used in each case is 4.5 nM. N.S., not significant. Full size image We next performed dual-colour imaging of dynein–GFP and p150 Glued 1-CC1-TMR on microtubules. Although isolated dynein–GFP co-purifies with dynactin ( Fig. 1b ), recombinant exogenously added p150 Glued 1-CC1-TMR was added in excess and effectively displaced endogenous dynactin as we observed co-localization ( Fig. 2e ) and co-migration of the co-complex ( Fig 2f , Supplementary Movie 2 ). The double-labelled dynein-GFP and 1-CC1-TMR complex exhibited both processive and diffusive motility along the microtubule, with a mean run length of 2.5±0.13 μm ( n =35), consistent with previous reports [8] , [12] . Importantly, in the presence of exogenous p150 Glued 1-CC1-TMR the recruitment of dynein molecules onto the microtubule was significantly enhanced ( Fig. 2g ), with a greater than 4-fold increase in binding events ( P <0.001, Fig. 2g,h ). To test whether the microtubule-binding activity of p150 Glued was necessary for this increased recruitment, we generated a recombinant coiled-coil fragment (CC1-TMR) of p150 Glued that robustly binds to dynein ( Supplementary Fig. 2b,c ) but lacks the N-terminal residues encoding both the CAP-Gly and basic domains ( Fig. 2b ). Addition of CC1-TMR did not affect dynein recruitment to the microtubule ( Fig. 2g,h ), indicating that the microtubule-binding domains of p150 Glued are required for the enhanced binding observed. p150 Glued regulates the dynein-microtubule interaction p150 Glued 1-CC1 displayed a concentration-dependent effect on dynein. This is shown in the maximum-intensity projections over time of dynein–GFP motility along the microtubules ( Fig. 3a ). We quantified the per cent length of microtubules decorated by dynein–GFP in these projections and saw a progressive increase with increasing concentrations of p150 Glued 1-CC1 ( Fig. 3b ). This effect of p150 Glued 1-CC1 could be due to an increase in the landing frequency of dynein or a decrease in the rate of detachment of dynein from microtubules, or both effects could potentially contribute. To address this, we measured the landing frequencies of dynein–GFP in the absence and presence of 1-CC1, and observed a 2.5-fold increase induced by the p150 Glued construct ( P <0.001, Fig. 3c ). To test for an effect on detachment, we rigor bound dynein–GFP to microtubules in the absence of ATP, and then flowed 5 mM Mg-ATP into the chamber to release the motors [28] . In the absence of 1-CC1, we observed rapid detachment of dynein induced by ATP. However, in the presence of p150 Glued 1-CC1, the dynein molecules remained bound to the microtubule for longer periods of time, suggesting that the motor is effectively tethered onto the microtubule via the microtubule-binding domains of dynactin at saturating ATP concentrations ( Fig. 3d,e ). Thus, we conclude that p150 Glued effectively recruits and retains dynein motors on microtubules by functioning as a dynamic tether. 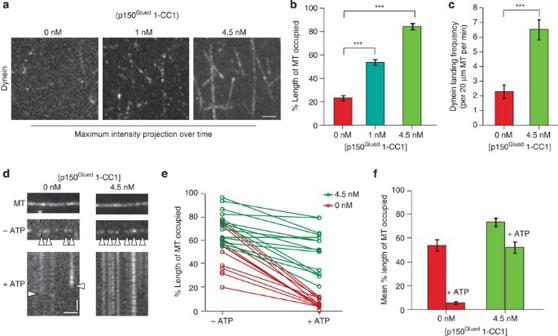Figure 3: p150Gluedregulates the association and dissociation of dynein from microtubules. (a) Maximum-intensity projection over time of dynein motility (movies recorded for 2 min) in the presence of p150Glued1-CC1. Horizontal bar, 2 μm. (b) Quantitation of the per cent occupancy of microtubules using line-scan intensity analysis. Mean±s.e.m.,n=20, two independent experiments, ***P<0.001, one-way analysis of variance with Tukey’spost-hoctest. (c) Addition of p150Glued1-CC1 increases the landing frequency of dynein. Mean±s.e.m.,n=20, two independent experiments, ***P<0.001, Student’st-test. (d) Representative images of dynein bound to microtubules in the absence of ATP and kymographs following 5 mM Mg-ATP wash. Horizontal bar, 2 μm. Vertical bar, 10 s. (e) Quantitation of the per cent occupancy of microtubules before and after the ATP wash. The corresponding data points for the same microtubules before and after the ATP wash are connected by a line,n=15 for each condition, two independent experiments. (f) Average of the data shown ine. The control had a 10-fold change post ATP wash while the addition of p150Glued1-CC1 reduced the change to ~1.5-fold. ***P<0.001, Student’st-test. Figure 3: p150 Glued regulates the association and dissociation of dynein from microtubules. ( a ) Maximum-intensity projection over time of dynein motility (movies recorded for 2 min) in the presence of p150 Glued 1-CC1. Horizontal bar, 2 μm. ( b ) Quantitation of the per cent occupancy of microtubules using line-scan intensity analysis. Mean±s.e.m., n =20, two independent experiments, *** P <0.001, one-way analysis of variance with Tukey’s post-hoc test. ( c ) Addition of p150 Glued 1-CC1 increases the landing frequency of dynein. Mean±s.e.m., n =20, two independent experiments, *** P <0.001, Student’s t -test. ( d ) Representative images of dynein bound to microtubules in the absence of ATP and kymographs following 5 mM Mg-ATP wash. Horizontal bar, 2 μm. Vertical bar, 10 s. ( e ) Quantitation of the per cent occupancy of microtubules before and after the ATP wash. The corresponding data points for the same microtubules before and after the ATP wash are connected by a line, n =15 for each condition, two independent experiments. ( f ) Average of the data shown in e . The control had a 10-fold change post ATP wash while the addition of p150 Glued 1-CC1 reduced the change to ~1.5-fold. *** P <0.001, Student’s t -test. Full size image Motility of p150 Glued in cell extracts is dynein-dependent To further dissect the domains of p150 Glued that are critical for the regulation of dynein motility, we sought to develop a more versatile single molecule assay. We performed motility assays using Halo-tagged constructs expressed in cell extracts ( Fig. 4a ). Similar assays have been used extensively to study kinesin motors and their regulation [29] , [30] , [31] but have not yet been applied to the dynein motor to test the function of its adaptors and cofactors like dynactin. 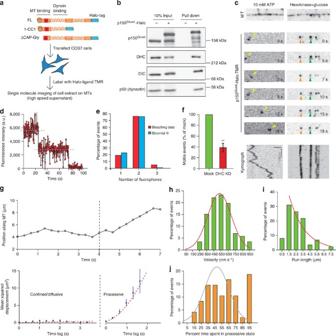Figure 4: The motility of p150Gluedin cell extracts is dynein driven and ATP dependent. (a) Schematic of the experimental design with an illustration of p150Gluedconstructs. (b) COS7 cell extracts were precipitated with a HaloLink resin that binds specifically to the Halo tag. Protein complexes bound to the resin were analyzed by immunoblotting. The dynein complex co-precipitates with p150Glued-Halo and the addition of the Halo tag at the C terminus does not interfere with the incorporation of p150Gluedinto the dynactin complex (as shown by p50). (c) Representative time series and corresponding kymographs of the motility of p150Glued-Halo in 10 mM Mg-ATP and in the presence of hexokinase and glucose (an ATP depletion system). Horizontal bar, 2 μm. Vertical bar, 5 s. All images are contrast inverted. (d) A representative time course of photobleaching of TMR-labelled p150Gluedshows two decay steps. Grey lines indicate the steps. (e) Frequency distribution of the photobleaching steps forn=42 particles fit with a binomial distribution. (f) Quantitation of the number of active, motile events of p150Glued-Halo in the mock and dynein knock-down conditions. The number of events was normalized to the length of the microtubules and the expression levels of p150Glued-Halo in extracts (densitometry analysis using ImageJ). DHC knockdown resulted in a reduction in the number of motile events. Mean±s.e.m.,n=3 experiments, **P<0.01, Student’st-test. (g) A representative trajectory of p150Glued-Halo with its corresponding MSD analysis. Error bars indicate s.e.m. (h,i) Velocity and run length distribution of the tracked p150Gluedparticles. Tracks (n=60, three independent experiments) were parsed into processive and diffusive states of motion using GrAND and velocities were calculated for the processive segments only. Curved lines indicate Gaussian and exponential decay fit, respectively. (j) Frequency distribution for the amount of time p150Glued-Halo spent in a processive state. Two populations can be observed—about 20% that are processive throughout the motion along the microtubule and the remaining that display both processive and diffusive phases. A Gaussian fit (shown in grey) excluding the last data point improves theR2from 0.45 to 0.81, suggesting there could be two populations. Figure 4: The motility of p150 Glued in cell extracts is dynein driven and ATP dependent. ( a ) Schematic of the experimental design with an illustration of p150 Glued constructs. ( b ) COS7 cell extracts were precipitated with a HaloLink resin that binds specifically to the Halo tag. Protein complexes bound to the resin were analyzed by immunoblotting. The dynein complex co-precipitates with p150 Glued -Halo and the addition of the Halo tag at the C terminus does not interfere with the incorporation of p150 Glued into the dynactin complex (as shown by p50). ( c ) Representative time series and corresponding kymographs of the motility of p150 Glued -Halo in 10 mM Mg-ATP and in the presence of hexokinase and glucose (an ATP depletion system). Horizontal bar, 2 μm. Vertical bar, 5 s. All images are contrast inverted. ( d ) A representative time course of photobleaching of TMR-labelled p150 Glued shows two decay steps. Grey lines indicate the steps. ( e ) Frequency distribution of the photobleaching steps for n =42 particles fit with a binomial distribution. ( f ) Quantitation of the number of active, motile events of p150 Glued -Halo in the mock and dynein knock-down conditions. The number of events was normalized to the length of the microtubules and the expression levels of p150 Glued -Halo in extracts (densitometry analysis using ImageJ). DHC knockdown resulted in a reduction in the number of motile events. Mean±s.e.m., n =3 experiments, ** P <0.01, Student’s t -test. ( g ) A representative trajectory of p150 Glued -Halo with its corresponding MSD analysis. Error bars indicate s.e.m. ( h , i ) Velocity and run length distribution of the tracked p150 Glued particles. Tracks ( n =60, three independent experiments) were parsed into processive and diffusive states of motion using GrAND and velocities were calculated for the processive segments only. Curved lines indicate Gaussian and exponential decay fit, respectively. ( j ) Frequency distribution for the amount of time p150 Glued -Halo spent in a processive state. Two populations can be observed—about 20% that are processive throughout the motion along the microtubule and the remaining that display both processive and diffusive phases. A Gaussian fit (shown in grey) excluding the last data point improves the R 2 from 0.45 to 0.81, suggesting there could be two populations. Full size image We expressed p150 Glued -Halo in COS7 cells and co-precipitated extracts with HaloLink resin. p150 Glued -Halo was incorporated into dynactin, as assessed by co-precipitation of the endogenously expressed dynactin subunit, dynamitin (p50; Fig. 4b ). Importantly, Halo-tagged p150 Glued co-precipitated both the heavy chain and intermediate chain of cytoplasmic dynein, indicating a robust interaction with endogenous dynein ( Fig. 4b ). Photobleaching analysis of the bound TMR ligand shows two decay steps and is well fit by a binomial distribution, consistent with the efficient dimerization of p150 Glued ( Fig. 4d,e ). We generated clarified cell extracts from COS7 cells expressing Halo-tagged p150 Glued constructs and performed single molecule assays tracking the motility of dynactin along microtubules ( Fig. 4c ). The observed motility closely resembled that observed for purified dynein–dynactin complexes ( Supplementary Movie 3 ) characterized by frequent switches from processive to diffusive motion. The observed motility is ATP- and dynein-dependent, as it was arrested by depletion of ATP from the flow chamber by hexokinase and glucose ( Fig. 4c ) and significantly reduced by depletion of dynein heavy chain from the cells by siRNA ( Fig. 4f and Supplementary Fig. 3a,b ). A representative trajectory parsed into segments using GrAND analysis along with the corresponding MSD analysis ( Fig. 4g ) shows that the motion switches from a confined/diffusive state to a processive state. We obtained velocities and run lengths for the processive segments of all particles tracked ( Fig. 4h,i ). The velocities obtained are comparable to those measured for isolated dynein–dynactin complexes ( Fig. 4h compared to Fig. 1e ). We also acquired data at higher frame rates (10 frames per second) and observed similar characteristics of motility ( Supplementary Fig. 3c ). For particles that had at least one processive segment, we generated a frequency distribution for the fraction of time spent in a processive state ( Fig. 4j ). In close agreement with the motility characteristics observed for isolated dynein–dynactin complexes ( Fig. 1g ), about ~20% of the p150 Glued -Halo-TMR particles tracked were processive throughout their motion along the microtubule while the remainder exhibited stochastic switching between processive and diffusive states. The average diffusion coefficient obtained from the diffusive phases was 0.055 μm 2 s −1 , consistent with previous reports [8] , [23] , [24] . Together, these results indicate that we have established a robust assay to study the properties of the dynein motor in complex with its adaptor dynactin; this assay will be useful in exploring the effects of other dynein adaptors in future. Using the cell extract assay, we asked whether the entire dynactin complex was required to increase the processivity of mammalian cytoplasmic dynein, as suggested by studies in a yeast strain lacking the Arp1 subunit of dynactin [12] , or whether the 1-CC1 construct of p150 Glued is sufficient to mediate these effects as suggested by our work with the purified recombinant fragment. p150 Glued 1-CC1-Halo expressed in COS7 cells extracts is sufficient to bind to dynein, but does not incorporate into the dynactin complex ( Supplementary Fig. 4a ). However, the motility we observed with p150 Glued 1-CC1-Halo was indistinguishable from that observed with full-length p150 Glued , as shown in a representative trajectory in Supplementary Fig. 4b ( Supplementary Movie 4 ). We observed no significant differences in the velocity or run length distribution (2.6±0.15 μm for p150 Glued versus 2.1±0.12 μm for p150 Glued 1-CC1) of the two constructs, or in the fraction of time spent in a processive state ( Supplementary Fig. 4c–e ). These observations suggest that incorporation of p150 Glued into the dynactin complex does not affect velocity or further enhance run lengths of the motor complex. Thus, we focused on the specific functions of the microtubule-binding domains of p150 Glued in activating dynein using our cell extract assay. The CAP-Gly domain of dynactin enhances dynein engagement Both the tandem CAP-Gly and basic domains in the N terminus of p150 Glued interact with microtubules [8] . To independently study the contribution of each of these domains to the motility of dynein, we compared the effects of two constructs—ΔCAP-Gly and Δ5-7. Δ5-7 is a naturally existing isoform of p150 Glued , which lacks three short exons (5, 6 and 7) and thus has a shorter basic domain compared with full-length p150 Glued ( Fig. 5a ). Representative kymographs comparing the motility of the ΔCAP-Gly and Δ5-7 constructs with full-length p150 Glued are shown in Fig. 5b . We observed no significant differences in the runs of the Δ5-7 isoform as compared with the full-length p150 Glued ( Supplementary Fig. 5a , 2.1±0.14 μm versus 2.6±0.15 μm). In contrast, runs observed with the ΔCAP-Gly construct were significantly faster, approximately 2-fold the rates were observed with the other two constructs ( P <0.001, Fig. 5c , Supplementary Fig. 5b ). Strikingly, binding times for the ΔCAP-Gly construct were extremely short ( Supplementary Movie 5 ). Histograms of time bound on microtubules for all particles tracked revealed that 70% of the ΔCAP-Gly particles were bound to microtubules for <10 s ( Fig. 5d ). Exponential decay fits to the cumulative frequency distribution curves for binding time of the full length, and ΔCAP-Gly constructs reveal a 3-fold higher detachment rate in the absence of the CAP-Gly domain ( Supplementary Fig. 5c ). Together, these data indicate that the CAP-Gly domain may function as an ATP-independent brake, as previously suggested from studies in which the CAP-Gly domain was non-specifically adsorbed to beads [8] , and that this activity both prolongs the microtubule interaction time of the dynein–dynactin complex and slows the motor during processive motility. 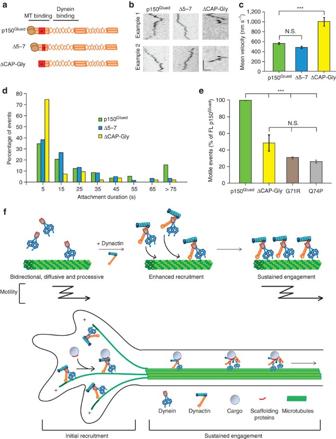Figure 5: The CAP-Gly domain of dynactin enhances the engagement of dynein onto microtubules. (a) Schematic of the Δ5-7 and ΔCAP-Gly constructs of p150Glued. While the Δ5-7 lacks much of the basic domain, ΔCAP-Gly is a deletion of the CAP-Gly domain. (b) Representative kymographs of the motility of p150Glued, Δ5-7 and ΔCAP-Gly constructs in complex with dynein along microtubules. Horizontal bar, 2 μm. Vertical bar, 5 s. Kymographs are contrast inverted. (c) Mean velocities of all the particles tracked for p150Glued, Δ5-7 and ΔCAP-Gly. Mean±s.e.m.,n=60 for p150Gluedand Δ5-7,n=40 for ΔCAP-Gly, three independent experiments, ***P<0.001, one-way analysis of variance with Tukey’spost-hoctest. (d) Frequency distribution of the binding times of Δ5-7 and ΔCAP-Gly in comparison to p150Glued. Greater than 70% of the ΔCAP-Gly particles have a binding time of less than 10 s (n=60 for each, three independent experiments). (e) Quantitation of the number of active, motile events of the ΔCAP-Gly and the two mutants G71R and Q74P in comparison to the full-length p150Glued. The number of events was normalized to the length of the microtubules and the expression levels of constructs in cell extracts (densitometry analysis using ImageJ). Mean±s.e.m.,n=3 independent experiments, ***P<0.001, one-way analysis of variance with Tukey’spost-hoctest. (f) Model for the regulation of dynein by dynactin depicting two functions of dynactin—initial recruitment and sustained engagement of the dynein motor. N.S., not significant. Figure 5: The CAP-Gly domain of dynactin enhances the engagement of dynein onto microtubules. ( a ) Schematic of the Δ5-7 and ΔCAP-Gly constructs of p150 Glued . While the Δ5-7 lacks much of the basic domain, ΔCAP-Gly is a deletion of the CAP-Gly domain. ( b ) Representative kymographs of the motility of p150 Glued , Δ5-7 and ΔCAP-Gly constructs in complex with dynein along microtubules. Horizontal bar, 2 μm. Vertical bar, 5 s. Kymographs are contrast inverted. ( c ) Mean velocities of all the particles tracked for p150 Glued , Δ5-7 and ΔCAP-Gly. Mean±s.e.m., n =60 for p150 Glued and Δ5-7, n =40 for ΔCAP-Gly, three independent experiments, *** P <0.001, one-way analysis of variance with Tukey’s post-hoc test. ( d ) Frequency distribution of the binding times of Δ5-7 and ΔCAP-Gly in comparison to p150 Glued . Greater than 70% of the ΔCAP-Gly particles have a binding time of less than 10 s ( n =60 for each, three independent experiments). ( e ) Quantitation of the number of active, motile events of the ΔCAP-Gly and the two mutants G71R and Q74P in comparison to the full-length p150 Glued . The number of events was normalized to the length of the microtubules and the expression levels of constructs in cell extracts (densitometry analysis using ImageJ). Mean±s.e.m., n =3 independent experiments, *** P <0.001, one-way analysis of variance with Tukey’s post-hoc test. ( f ) Model for the regulation of dynein by dynactin depicting two functions of dynactin—initial recruitment and sustained engagement of the dynein motor. N.S., not significant. Full size image Multiple mutations in the CAP-Gly domain of p150 Glued are causative for neurodegenerative diseases. A G59S mutation that lies at the core of the folded CAP-Gly domain induces misfolding and aggregation, leading to motor neuron-degeneration [19] , [21] . A series of nearby mutations that are surface-exposed within the microtubule-binding domain cause a distinct disease—a lethal variant of parkinsonism known as Perry syndrome. We examined two Perry-associated mutations, G71R and Q74P in our assay, and found that both mutations phenocopy the ΔCAP-Gly construct. All constructs were expressed to a similar degree in our cell extracts ( Supplementary Fig. 5d ) but the G71R, Q74P and ΔCAP-Gly constructs all showed significantly decreased motile events as compared with full-length p150 Glued ( Fig. 5e ). Together, these results indicate that the CAP-Gly domain has a dual effect. It promotes the sustained engagement of the motor on microtubules by acting as a tether, an activity abrogated by the Perry mutations. However, through its tethering activity, the CAP-Gly domain can induce a drag on dynein, acting as a brake to slow the motor during motility along the microtubule and this function could potentially be regulated in the cell. Dynactin is a key adaptor for the cytoplasmic dynein motor and every organism that has cytoplasmic dynein has dynactin as well [32] . Although a role for dynactin in increasing the processivity of dynein has been previously proposed, the functional significance of the microtubule-binding capacity of dynactin has remained controversial [10] , [13] , [14] , [15] , [16] , [17] , [23] . Here we used single molecule approaches and dual-colour total internal reflection fluorescence microscopy (TIRF) to definitively dissect the functional role that dynactin plays in dynein-driven motility. We isolated GFP tagged dynein from a knock-in mouse line and used purified recombinant p150 Glued constructs to examine this problem. We found that dynactin significantly enhances the recruitment of dynein onto microtubules and the microtubule-binding capacity of dynactin is required for this recruitment. Dynactin increases the landing frequency and decreases the detachment rate of dynein from microtubules. We also demonstrate that in contrast to data from yeast [12] , the p150 Glued C terminus is not required for this activity. Further dissection of the N terminus of p150 Glued indicates that the CAP-Gly domain is key in promoting the sustained interaction of the dynein motor with microtubules. Importantly, point mutations in the CAP-Gly domain associated with Perry syndrome phenocopy the deletion of CAP-Gly in our assays. These in vitro observations are in strong agreement with recent studies in Drosophila and mammalian neurons, which demonstrated that the CAP-Gly domain of dynactin is important for the initiation of dynein-driven transport of cargos from the distal end of the axon and suggest that this function is perturbed in neurodegenerative disease [16] , [17] . Our results are strikingly different from the yeast dynein–dynactin system in that the microtubule-binding capacity of Nip100 (yeast homologue for p150 Glued of dynactin) is dispensable in increasing the processivity of dynein [12] . There is also evidence for the lack of interaction of Nip100 with microtubules [12] , which is in contrast to the robust interaction of p150 Glued with microtubules [9] . Further, there is growing evidence that yeast dynein is fundamentally different from the mammalian dynein. Yeast dynein is a slower and stronger motor that takes occasional backward steps, while mammalian dynein is a weaker and faster motor with frequent backward runs and interspersed periods of diffusion [23] , [24] , [33] , [34] . Given these important differences, we suggest that the molecular mechanisms of dynactin described here have specifically evolved in higher eukaryotes. Motor-driven transport involves three key steps—initial recruitment of the motor–cargo complex, transport along cytoskeleton tracks and the off-loading of the cargo at its destination. Thus, the question remains: what is the specific function of dynactin in dynein-driven transport? And is the function of dynactin regime-specific: single motor versus multiple motors; low load versus high load? In small cells with bundled microtubules, the trafficking defects caused by p150 Glued knockdown can be rescued with a construct lacking the microtubule-binding domain [14] , [15] . Trafficking of organelles along the stable and densely packed microtubules of the axon shaft also does not require the CAP-Gly domain [17] . However, for other cellular functions, the CAP-Gly domain is required [13] , [14] . Thus, we propose that the CAP-Gly domain of dynactin becomes essential in specific instances of dynein-driven transport ( Fig. 5f ). We propose three specific cases where the microtubule-binding capacity of dynactin is necessary to enhance dynein function: (1) For small cargoes with very few dynein motors, dynactin can actively maintain an interaction with the microtubule during detachment of both dynein heads leading to sustained motility. (2) For large cargoes which generate a high load for the motors, the CAP-Gly domain enhances the ability of dynein to produce movement [13] . (3) Transport of cargos along individual, dynamic microtubules [35] such as those in the axon terminal as opposed to stable, densely packed or bundled microtubules. Importantly, initial recruitment of dynein motor–cargo complex often occurs near the cell periphery where highly dynamic microtubule plus ends are enriched. Given the dynamic and crowded cellular environment, all of these are regimes in which the dynein motor must work effectively. Thus, our results converge to a model wherein dynactin is required for the recruitment of the dynein motor onto microtubules for efficient initiation of transport and further, the CAP-Gly domain of dynactin functions as both tether and brake to promote the engagement of dynein on the microtubule. Reagents Cytoplasmic dynein was purified from mice ( Mus musculus ) that are homozygous knock-in for DIC1 replaced with DIC1–eGFP–3X FLAG. All animal protocols were approved by the Institutional Animal Care and Use Committee (IACUC) at the University of Pennsylvania. Both male and female young adult mice (4–8 months old) were used. All p150 Glued constructs were generated from the human DCTN1 sequence (GenBank accession number NM_004082 ). The Halo tag from the pHTC Halo tag CMV-neo vector (Promega) was fused in-frame to the C terminus of the p150 Glued constructs and cloned into pcDNA3 vector. DNA constructs encoding the Perry syndrome point mutations were obtained from M. Farrer. p150 Glued 1-CC1 includes amino acid residues up to Q547 and the ΔCAP-Gly construct starts from K115. Monoclonal antibodies to p150 (610474, 1:5,000), p50 (611003, 1:1,000) and β-catenin (610153, 1:5,000) were from BD Transduction Laboratories, monoclonal antibodies to actin (1501R, 1:10,000); and DIC (MAB1618, 1:1,000) were from Millipore; and monoclonal antibody to Halo tag (G9211, 1:1,000) was from Promega. A polyclonal antibody to dynein heavy chain (R-325, 1:250) was from Santa Cruz. Uncropped Western blots are shown in Supplementary Fig. 6 . For binding experiments, monoclonal antibody to FLAG (clone M2, 1:10) from Sigma and monoclonal tetra-His antibody from Qiagen (34670, 1:10) were used. For RNA interference (RNAi) knockdown of dynein, 50 nM of the short interfering RNA (siRNA) duplex (Dharmacon) against human dynein heavy chain (GenBank accession number NM_001376 ; 5′-GAGAGGAGGUUAUGUUUAAUU-3′) was used. Protein purification and binding assays Cytoplasmic dynein was purified from brain tissue from adult mice by microtubule affinity and ATP release, followed by sucrose density gradient centrifugation as described [36] . Briefly, adult mouse brain tissue was homogenized at 1:1 weight/volume in chilled motility assay buffer (10 mM PIPES, 50 mM potassium acetate, 4 mM MgCl 2 , 1 mM EGTA, pH 7.0 with KOH) with 1 mM dithiothreitol (DTT), 0.5 mM Mg-ATP and protease inhibitors (2 mM phenylmethylsulfonyl fluoride, 0.02 mg ml −1 Tosyl arginine methyl ester (TAME), 0.02 mg ml −1 leupeptin, 0.002 mg ml −1 pepistatin-A). Hexokinase (1 U ml −1 ) and 1 mg ml −1 glucose were used for microtubule affinity and 20 mM Mg-ATP was used for microtubule release. The supernatant from the microtubule release was fractionated on a 5–25% continuous sucrose density gradient and 1 ml fractions were collected and analyzed by SDS–PAGE and Western blotting. p150 Glued 1-CC1-Halo-Flag (amino acids 1–547 of DCTN1 , NM_004082) was expressed in Sf9 cells using baculovirus following standard methods. After harvest, cells were lysed in Buffer A (Tris-buffered saline supplemented with 200 mM NaCl, 10% glycerol, 0.5% igepal, 0.01 mg ml −1 TAME, 0.01 mg ml −1 leupeptin and 1 mM PMSF) in a Dounce homogenizer. After clarification, protein was captured on an M2 agarose column (Sigma), and further purified on a MonoS column (GE Healthcare) with buffer A as above and buffer B as Tris-buffered saline supplemented with 10% glycerol and 1 M KCl. Peak fractions were incubated with Halo tag TMR Ligand (Promega) overnight at 4 °C, then separated from unreacted dye on a Superdex column (GE Healthcare) in BRB80 (80 mM PIPES, 1 mM MgCl 2 , 1 mM EGTA, pH 6.8 with KOH) supplemented with 200 mM KCl and 10% glycerol. Peak fractions were combined, aliquoted and flash frozen and stored in liquid nitrogen. p150 Glued CC1-Halo-6xHis (amino acids 216–547 of DCTN1 , NM_004082) was inserted into pET-29b (Novagen). For expression, transformed Rosetta E.coli (Novagen) were grown in LB at 37 °C at 325 r.p.m. under standard kanamycin selection. At OD 600 ~0.7, cultures were transferred to 25 °C and induced with 0.5 mM isopropyl-β-D-thiogalactoside. After 16 h, cells were harvested and resuspended in His-binding buffer (500 mM NaCl, 20 mM Tris-HCl, pH 7.8, 15 mM imidazole, 1 mM Tris(2-carboxyethyl)phosphine hydrochloride (TCEP), 0.01 mg ml −1 TAME, 0.01 mg ml −1 leupeptin, and 1 mM PMSF). Cells were then lysed by French press (Thermo) at 18,000 psi followed by DNAse I and RNAse H treatment (Roche). The lysate was clarified at 45,000 g for 20 min at 4 °C. The supernatant was filtered and loaded onto a 1 ml HisTrap column (GE Healthcare) by fast protein liquid chromatography. The column was washed with binding buffer and then eluted with binding buffer supplemented with 0.5 M imidazole. The peak fraction was incubated overnight a 4 °C with 5 mM TMR ligand. The protein was run on a Superdex column (GE Healthcare) pre-equilibrated with BRB80 supplemented with 200 mM KCl and 10% glycerol. Peak fractions were combined, aliquoted, flash frozen and stored in liquid nitrogen. Binding assays of purified proteins (p150 Glued 1-CC1 and p150 Glued CC1) with dynein was performed by first incubating the proteins with protein G dynabeads (Life Technologies) coated with either anti-FLAG antibody or anti-His antibody, followed by the addition of dynein purified from bovine brain supplemented with 1 mg ml −1 bovine serum albumin. The proteins were eluted off the beads in denaturing buffer and the presence of dynein in the eluate was assayed by Western blot. Cell culture, transfections and pull downs COS7 cells (ATCC, CRL-1651) were cultured in DMEM with glutamax and 10% foetal bovine serum. Cells were transiently transfected with Fugene 6 (Roche) according to manufacturer’s instructions; cells were harvested 18–24 h post transfection. For RNAi knockdown, cells were transfected with siRNA duplexes using Lipofectamine RNAiMax (Invitrogen) with optimal knockdown obtained between 40 and 48 h. Immunoblots for knock-down experiments were analyzed by densitometry using ImageJ (NIH). For pull down assays using HaloLink resin (Promega), cells were lysed in 50 mM HEPES, 25 mM NaCl, 1 mM EDTA, 1 mM MgCl 2 , pH 7.0 with 1 mM DTT, 0.5% triton X-100 and protease inhibitors (1 mM PMSF, 0.01 mg ml −1 TAME, 0.01 mg ml −1 leupeptin and 0.001 mg ml −1 pepistatin-A). Lysates were incubated with the resin for 2 h at 4 °C and washed according to the manufacturer’s instructions. Precipitated proteins were analyzed by SDS–PAGE and Western Blotting. Single molecule motility assays Motility assays were performed in flow chambers made with glass slides and silanized (PlusOne Repel Silane, GE Healthcare) coverslips attached together using adhesive tape, forming a chamber with a volume of 10 μl. There was a 5 min incubation time between each solution that was flowed into the chamber. The chamber was first incubated with 10 μl of 1:50 dilution of the monoclonal anti-tubulin antibody (Sigma), then blocked with two chamber volumes of 5% pluronic F-127 (sigma). Labelled (either Rhodamine or Alexa 488) taxol-stabilized microtubules were flowed into the chamber and allowed to bind to the anti-tubulin antibody. Finally, purified protein or cell extract was flowed in with Mg-ATP (1 mM for purified proteins and 10 mM for cell extract), 1 mg ml −1 bovine serum albumin, 1 mg ml −1 casein, 20 μM taxol, 1 mM DTT and an oxygen scavenging system [37] . For photobleaching experiments ATP was depleted with 1 U ml −1 hexokinase and 1 mg ml −1 glucose and the oxygen scavenging system was omitted to allow for complete photobleaching. For motility assays with dynein–GFP and purified p150 Glued 1-CC1-TMR, dynein was incubated with p150 Glued 1-CC1 for 5 min at room temperature for co-complex formation before flowing into the chamber. For all co-migration experiments, 7-amino-4-methyl coumarin-3-acetic acid (AMCA)-labelled tubulin (cytoskeleton) was used to prepare taxol-stabilized microtubules. For motility assays with cell extracts, COS7 cells 18–24 h post transfection were incubated with Halo ligand TMR (Promega) following manufacturer’s instructions. The cells were then lysed in 40 mM HEPES, 1 mM EDTA, 120 mM NaCl, 0.1% Triton X-100, 1 mM Mg-ATP supplemented with protease inhibitors (same as above). The lysate was clarified by centrifugation at 1,000 g first and then 100,000 g . The extract was diluted in P12 buffer (12 mM PIPES, 1 mM EGTA, 2 mM MgCl 2 , pH 6.8) right before perfusion into the flow chamber. For a 70–80% confluent 6 cm plate, cells were lysed in 50 μl lysis buffer, which was then diluted 1:100 for single molecule imaging. All movies were acquired at room temperature at 3 or 10 frames per second as noted, except for dual-colour co-migration experiments that was imaged at 1 frame per second, using a Nikon TIRF system (Perkin Elmer) on an inverted Ti microscope with the × 100 objective and an ImagEM C9100-13 camera (Hamamatsu Photonics) controlled by Volocity software. Particle tracking and data analysis Particle tracking was performed using the TrackMate plugin in Fiji [38] . Particles that ran into other adjacent particles, hit the microtubule ends repeatedly or were on microtubule bundles, were excluded from analysis. Only particles with trajectories that could be clearly visualized were tracked and analyzed, and each track detected by TrackMate was confirmed by visual inspection. The tracking resolution was determined to be 36 nm, obtained from the standard deviation of the tracking of stationary particles on microtubules. As the motility of dynein frequently switches from processive to diffusive states, we developed a new algorithm, GrAND to parse these states within a given track. Each track was split into stationary and non-stationary segments using approximately three times the tracking error (100 nm) as a threshold. The non-stationary segments were then smoothed using the locally weighted scatterplot smoothing (‘lowess’) function in MATLAB with the span (smoothing window) set to 20% of the track length. Twenty per cent was determined to be optimum for our acquisition rates and track lengths. The slope at each point of the smoothed track was obtained (gradient analysis) and points of zero slope were identified as nodes. These nodes are points dividing a given trajectory into smaller segments of constant velocity. Smoothing is done only to identify the nodes for a given track and all further analysis is done on raw data. Once the nodes were identified, MSD analysis was performed on the individual segments to classify them as processive or diffusive. Velocity and run length measurements were obtained for the processive segments only. Simulations To validate our GrAND method, we simulated tracks using parameters from our experimental data. These parameters include temporal resolution (3 frames per second), track duration (30 s—average track length of the dynein–GFP particles tracked), velocity (550 nm s −1 ), diffusion coefficient (0.055 μm 2 s −1 ) and noise (Gaussian distribution with mean ( μ )=0, standard deviation ( σ )=100 nm ( × 3 tracking error)). The inputs to the simulation include probability of diffusion ( P d ) and processive ( P p ) motions such that P d + P p =1. These probabilities indicate the fraction of time spent in diffusive and processive motion, respectively. For example, a particle in a track with a duration of 30 s (90 frames) having P d =2/3 and P p =1/3 would spend 20 s (60 frames) and 10 s (30 frames) in diffusive and processive motions, respectively. Since the motion of dynein frequently involves segments of processive motion interspersed with segments of diffusion, we first generated either diffusive or processive segments, which are then concatenated randomly to generate the whole track. In each case, the number of segments was set to five. For processive segments, the particle displacement is given by x = v × Δ t . For diffusive segments, the displacements were obtained from a normal distribution with μ =0, σ =square root (2 × D × Δ t ) nm. Photobleaching analysis To prevent dissociation of the particles from microtubules, data from motility assays in the presence of hexokinase and glucose were used to analyze photobleaching. Only particles bound to microtubules were analyzed. A 5 × 5 pixel region of interest was drawn around the particle and the intensity was recorded from each frame using the Plot Profile in FIJI. Another 5 × 5 pixel region of interest was drawn in the vicinity of the particle to record the background intensity. For each frame, the background was subtracted and the intensity was plotted with time to determine the number of bleaching steps. Landing events The dynein concentration was kept constant across experiments comparing different conditions ( Figs 2 and 3 ). To measure the number of landing events for dynein in the presence of p150 Glued 1-CC1, microtubules were randomly chosen from the centre of TIRF field and particles on the microtubules were scored by line-scan intensity analysis. Distinct and clear particles on the microtubules showed up as peaks in the intensity profile corrected for background (background intensity was obtained by drawing a line in the vicinity of the microtubule and recording the intensity). Each peak was visually inspected for the presence of a particle. The length of microtubules occupied was determined from the maximum-intensity projection over time of dynein in a similar way. Only intensities at least 10% above background were scored as occupied. In each case, the data was normalized to the length of the microtubule. For dynein landing frequency measurements in Fig. 3 , microtubules in the TIRF field were scored for motile events by kymograph analysis using Multiple Kymograph plugin in FIJI. For Fig. 3e , microtubules were randomly chosen in each condition and for each microtubule the dynein–GFP intensity was recorded before and after the ATP wash. The intensities were recorded by the line-scan intensity analysis in FIJI. Extracts from cells showing ≥85% dynein knockdown, as determined by densitometry analysis with ImageJ, were analyzed to test the dependence of p150 Glued motility on dynein. To measure landing events ( Figs 4h and 5e ), microtubules in the TIRF field were scored for motile events by kymograph analysis using Multiple Kymograph plugin in FIJI. The number of events was normalized to the length of the microtubules and the expression levels of p150 Glued -Halo were quantified by densitometry analysis using ImageJ (NIH). Statistical methods All statistics were performed in GraphPad Prism. Student’s t -test was used when comparing two data sets while one-way analysis of variance with Tukey’s post-hoc test was used with multiple data sets. How to cite this article: Ayloo, S. et al. Dynactin functions as both a dynamic tether and brake during dynein-driven motility. Nat. Commun. 5:4807 doi: 10.1038/ncomms5807 (2014).